Silver-catalysed direct amination of unactivated C–H bonds of functionalized molecules Carbon–nitrogen bond formation from inert C–H bonds is an ideal organic transformation and a highly desirable method for the synthesis of N-containing molecules due to its high efficiency and atom economy. In this report, we develop a general reaction to achieve an unprecedented selective intramolecular amination of unactivated C–H bond in the absence of complex directing groups. Functionalized heterocyclic products are built up from readily available linear amines through simple and reliable silver catalysis, representing a new silver-based C–H functionalization. This method displays preference for primary sp 3 C–H bonds and exhibits distinct chemo- and regioselectivity compared to existing methods of direct amination (Hofmann–Löffler–Freytag reaction and nitrene insertion). The study highlights the manipulation of unfunctionalized groups in organic molecules to furnish complex structural units in the natural and bioactive molecules. Direct functionalization of inert C–H bonds is of great importance with the potential to fundamentally change the strategy of organic synthesis [1] , [2] , [3] . This chemistry can directly convert simple, cheap and readily available raw materials into highly valuable and useful products by the manipulation of inert unfunctionalized groups [4] , [5] , [6] , [7] , [8] . The greatest challenge in this field is therefore to achieve the chemo- and regioselectivity in C–H functionalization among many C–H bonds in organic molecules, while keeping an array of functional groups intact. In addition to the issue of selectivity, there are more challenges toward the direct functionalization of sp 3 C–H bonds, including: their high bond dissociation energy, inaccessibility of the independent C–H bonding and antibonding orbitals as well as steric hindrance. In the past decades, great progress has been made in such fields to convert aliphatic sp 3 C–H bonds to C–C, C–O and C–B bonds in either stoichiometric or catalytic manner based on transition-metal catalysis [9] , [10] , [11] , [12] , [13] , [14] , [15] . The present article focuses on the direct amination of inert C sp3 –H bonds, especially primary C–H bonds to construct aza-heterocycles. Nitrogen-containing heterocycles, such as pyrrolidines, oxazolidines and tetrahydroquinolines, are dominant both in naturally occurring and man-made compounds, which often exhibit high levels of biological activity. In particular, the pyrrolidine and tetrahydroquinoline derivatives are privileged structural units in natural products and pharmaceuticals as exemplified by the structures of strychnine, folicanthine and mesembrine and so on ( Fig. 1a ) [16] , [17] , [18] , [19] , [20] . Many chemists have devoted themselves to searching for practical and convenient synthetic methods for accessing such ubiquitous structural units by direct oxidative amination of C–H bonds [21] , [22] , [23] , [24] , [25] , [26] , [27] , [28] , [29] , [30] , [31] , [32] , [33] , [34] , [35] , [36] , [37] , [38] . In fact, efforts toward such a goal can be traced back to the historical Hofmann–Löffler–Freytag reaction in early 19th century and its advanced versions-the Baldwin and Doll modification and the Suárez modification [21] , [22] , [23] , [24] , [25] , [26] , [27] , [28] , [29] . Another effective method for approaching direct amination of sp 3 C–H bonds is to utilize nitrene insertion via transition-metal catalysis ( Fig. 1b ) [30] , [31] , [32] , [33] . Amongst these, silver complexes were first founded to promote the nitrene insertion [34] , [35] . Recently, Hennessy and Betley [36] developed a successful example for carrying out such transformation via Fe catalysis under mild conditions. The power of this strategy has also been demonstrated in the synthesis of the natural product tetrodotoxin [37] . 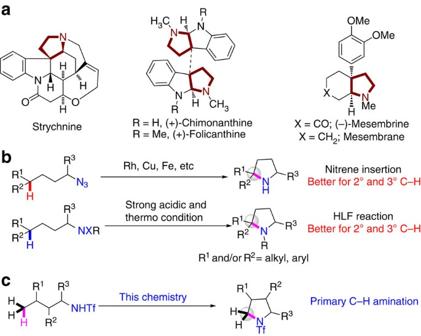Figure 1: Pyrroline structural active compounds and synthetic methods. (a) Diversified structures of alkalines containing semi-unsubstituted pyrroline structural units. (b) Secondary and tertiary aliphatic C–H amination through transition-metal catalyzed nitrene insertion and Hofmann–Löffler–Freytag reaction (HLF reaction). (c). Rational design on direct primary C–H amination via transition-metal catalysis. Figure 1: Pyrroline structural active compounds and synthetic methods. ( a ) Diversified structures of alkalines containing semi-unsubstituted pyrroline structural units. ( b ) Secondary and tertiary aliphatic C–H amination through transition-metal catalyzed nitrene insertion and Hofmann–Löffler–Freytag reaction (HLF reaction). ( c ). Rational design on direct primary C–H amination via transition-metal catalysis. Full size image Notably, the selectivity in these two elegant transformations is highly dependent on the nature of C–H bonds. In general, secondary and tertiary C–H bonds are much more reactive than the primary one for both reactions. Primary C–H bonds could be accessed only in cases of conformational bias [38] , [39] . To approach the primary selectivity of direct amination, Chen and Daugulis groups successfully developed a Pd-catalysed cyclization to specific ring systems by using a directing strategy while the manipulation of protecting group by multistep transformations limited its applications [40] , [41] , [42] . To achieve the primary selectivity to construct the abundant five-membered heterocyclic products from easily available amine derivatives without the requirement of complicated directing groups, new strategies and new catalytic systems are highly desirable [43] , [44] . Notably, the compatibility with an array of the functionalities, the availability of the starting materials and the reliability of the new reaction system are important for potential applications. Herein, we report an unprecedented Ag-catalysed direct amination of primary sp 3 C–H, secondary benzylic C–H and aryl C–H bonds from linear triflamide (1,1,1-trifluoromethanesulfonamide) under simple conditions. This represents a powerful approach to access structures widely existing in natural products and druggable molecules. C–H cyclizations We chose the sulphonamides as the substrates due to their easy availability and broad application in organic synthesis. After extensive screening of a variety of transition-metal catalysts, oxidants, bases and ligands, we found that the combination of AgOAc, K 2 CO 3 , 4,4′-di- t -butyl-2,2′-bipyridine and PhI(OTFA) 2 gave the best results and the desired pyrolidines were isolated from linear alkyltriflamide ( Supplementary Tables 1–3 ). This method was successfully applied to a variety of triflamide derivatives, providing the cyclized products in fair to good yields ( Fig. 2 ). Notably, the presence of substituents at the β-position is favourable for the transformation of products and good yields of 2a and 2b were obtained. α-Substitution decreased the yields and the examples indicate steric hindrance playing a key role in these annulations ( 2c – e ). γ-Substituted linear triflamide afforded the pyrrolidine product in a fair yield ( 2f ). Substrate 1g afforded 2g in a good yield with the expected preference for the trans isomer (86:14). 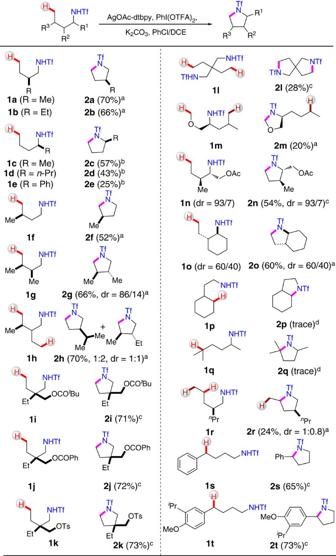Figure 2: Direct amination of primary and benzylic C–H bonds. The reaction scheme is shown above the table.aUnless otherwise noted, the reaction conditions were as follows: sulphonamide (0.25 mmol), AgOAc (20 mol%), PhI(OTFA)2(2.0 equiv), ligand (20 mol%), K2CO3(2.0 equiv), PhCl/dichloroethane (DCE) (1.5 ml/1.5 ml), 120 °C, 12 h. The isolated yield was shown in the parentheses.bSulphonamide (0.25 mmol), AgOAc (20 mol%), PhI(OTFA)2(2.0 equiv), ligand (20 mol%), K2CO3(4.0 equiv), PhF/Trichloroethane (1.5 ml/1.5 ml), 120 °C, 2 h; then another PhI(OTFA)2(2.0 equiv) was added and the reaction was continued for another 2 h.cSulphonamide (0.10 mmol), AgOAc (20 mol%), PhI(OTFA)2(2.0 equiv), ligand (20 mol%), K2CO3(2.0 equiv), PhCl/DCE (1.0 ml/1.0 ml), 120 °C, 12 h.dThe yield was determined by1H NMR of the crude reaction mixture. Figure 2: Direct amination of primary and benzylic C–H bonds. The reaction scheme is shown above the table. a Unless otherwise noted, the reaction conditions were as follows: sulphonamide (0.25 mmol), AgOAc (20 mol%), PhI(OTFA) 2 (2.0 equiv), ligand (20 mol%), K 2 CO 3 (2.0 equiv), PhCl/dichloroethane (DCE) (1.5 ml/1.5 ml), 120 °C, 12 h. The isolated yield was shown in the parentheses. b Sulphonamide (0.25 mmol), AgOAc (20 mol%), PhI(OTFA) 2 (2.0 equiv), ligand (20 mol%), K 2 CO 3 (4.0 equiv), PhF/Trichloroethane (1.5 ml/1.5 ml), 120 °C, 2 h; then another PhI(OTFA) 2 (2.0 equiv) was added and the reaction was continued for another 2 h. c Sulphonamide (0.10 mmol), AgOAc (20 mol%), PhI(OTFA) 2 (2.0 equiv), ligand (20 mol%), K 2 CO 3 (2.0 equiv), PhCl/DCE (1.0 ml/1.0 ml), 120 °C, 12 h. d The yield was determined by 1 H NMR of the crude reaction mixture. Full size image Substrate scope We further expanded the substrate scope containing heteroatom functional groups. To our satisfaction, we found that O-containing functional groups are well-tolerated ( 2i , 2j , 2k ). Remarkably, the excellent leaving group –OTs (4-toluylsulfonoxyl) was compatible. The spirocyclic 2l was obtained from substrate 1l through double cyclization, albeit in relatively low yield. The 1,2-amino alcohol derivative 1m afforded oxazolidine 2m , indicating the enhanced reactivity of the C–H bond adjacent to the heteroatom in spite that the reaction leaves much room for the improvement. The protected amino alcohol 1n well proceeded the cyclization, with the retention of the stereogenic centres, providing an efficient method to produce unnatural proline derivatives. The five–six fused-ring compound 2o was formed in a satisfactory yield, and the diastereoselectivity was controlled by the starting materials. Compared with primary C–H bonds, secondary or tertiary C–H bonds exhibit poor reactivity, which is distinct from Hofmann–Löffler–Freytag reactions or nitrene insertions, thus probably pointing out the different mechanistic pathway 1p and 1q (after 12 h, 59% of 1p and 51% of 1q were recovered). Moreover, five-membered ring is much favoured even in the presence of more reactive primary C–H bonds for the formation of six-membered ring (24% of the 1r was recovered). In contrast, the more reactive benzylic secondary C–H bonds in 1s and 1t could be addressed, expanding the scope for further applications. Due to the distinct proposed pathway of such an amination from previous methods, we envisioned that this chemistry could be applicable for direct amination of aromatic C–H bonds. Thus, we extended this chemistry to build up the structurally important tetrahydroquinoline scaffolds from 3-arylpropyl triflamide 3 ( Fig. 3 ). A series of γ-aryl substituted sulphonamides were examined and it was found that: (1) substituented aliphatic motifs at different positions do not obviously affect the efficiency; (2) electron-rich aromatics react preferentially; (3) compared with the inert primary sp 3 C–H bond, the sp 2 C–H bond on the aromatic ring is more reactive; and (4) notably, functionalized substrate 3h also exhibited good reactivity, thus indicating great potential for their applications. 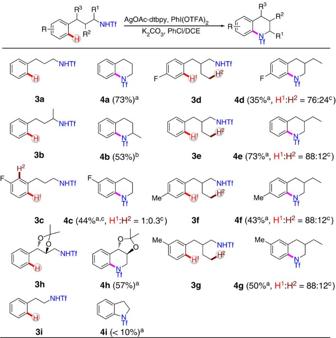Figure 3: Direct amination of aromatic C–H bonds. aUnless otherwise noted, the reaction conditions were as follows: sulphonamide (0.25 mmol), AgOAc (1.0 equiv), PhI(OTFA)2(2.0 equiv), ligand (20 mol%), K2CO3(2.0 equiv), PhCl/dichloroethane (DCE) (1.5 ml/1.5 ml), 120 °C, 12 h. The isolated yield was shown in the parentheses.bSulphonamide (0.25 mmol), AgOAc (1.0 equiv), PhI(OTFA)2(2.0 equiv), ligand (20 mol%), K2CO3(2.0 equiv), PhCl/DCE(1.0 ml/1.0 ml), 120 °C, 2 h; then another PhI(OTFA)2(2.0 equiv) was added and the reaction was continued for 2 h.cThe ratio was determined by crude1H NMR of the crude reaction mixture. Figure 3: Direct amination of aromatic C–H bonds. a Unless otherwise noted, the reaction conditions were as follows: sulphonamide (0.25 mmol), AgOAc (1.0 equiv), PhI(OTFA) 2 (2.0 equiv), ligand (20 mol%), K 2 CO 3 (2.0 equiv), PhCl/dichloroethane (DCE) (1.5 ml/1.5 ml), 120 °C, 12 h. The isolated yield was shown in the parentheses. b Sulphonamide (0.25 mmol), AgOAc (1.0 equiv), PhI(OTFA) 2 (2.0 equiv), ligand (20 mol%), K 2 CO 3 (2.0 equiv), PhCl/DCE(1.0 ml/1.0 ml), 120 °C, 2 h; then another PhI(OTFA) 2 (2.0 equiv) was added and the reaction was continued for 2 h. c The ratio was determined by crude 1 H NMR of the crude reaction mixture. Full size image Figure 6: Direct amination of linear amino acids derivatives. ( a ) Direct amination to produce substituted proline and tetrahydroquinolyl carboxylic acid derivatives from linear amino acids. 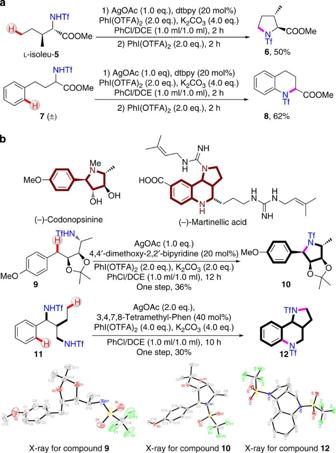Figure 6: Direct amination of linear amino acids derivatives. (a) Direct amination to produce substituted proline and tetrahydroquinolyl carboxylic acid derivatives from linear amino acids. (b) Applications to the synthesis of natural structural scaffolds. ( b ) Applications to the synthesis of natural structural scaffolds. Full size image Competition experiments Competition experiment between primary C–H bonds and secondary C–H bonds was carried out ( Supplementary Fig. 1 ). As predicted, the preference for amination is C Me –H>>C methylene −H ( Fig. 4a ). The KIE experiments have been conducted and we found that the intramolecular and intermolecular kinetic isotopic effect values at the benzylic position were 2.8 and 1.4, respectively ( Supplementary Figs 2 and 3 ). On the basis of all these results, we proposed that this transformation was preferred to a proton abstraction pathway. With the assistance of strong σ-donor chelating N-ligands, the silver complex could be oxidized to Ag(III) after the ligand exchange. The hyperelectrophilic Ag(III) centre attacks the less steric hindered the primary C–H bonds, followed by electrophilic deprotonation, which probably goes through a concerted metallation/deprotonation process in the presence of TFAO − (1,1,1-trifluoroacetate anion) as a base. Afterwards, the reductive elimination produced the desired product, releasing Ag(I) to fulfil the catalytic cycle ( Fig. 5 ). The steric and electronic outcomes based on different substrates are consistent with this hypothesis. 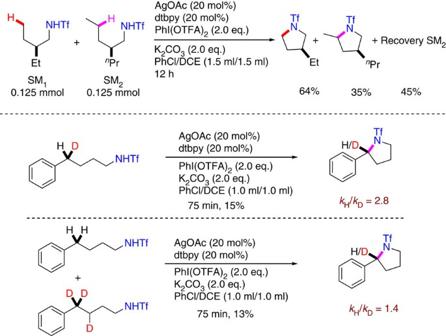In some cases, a small amount of the desired product is also observed in the absence of the Ag catalyst, indicating the competitive existing radical pathway, which may induce the low KIE in kinetic studies. Figure 4: Competition experiment and kinetic isotope effect. (a) Intermolecular competition experiment. (b) Intra/intermolecular kinetic isotope effect at benzylic position. Figure 4: Competition experiment and kinetic isotope effect. ( a ) Intermolecular competition experiment. 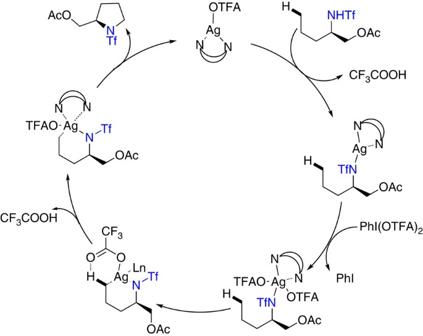( b ) Intra/intermolecular kinetic isotope effect at benzylic position. Figure 5: The proposed catalytic cycle of direct amination via Ag catalysis. A concerted metallation/deprotonation (CMD) process. Full size image Figure 5: The proposed catalytic cycle of direct amination via Ag catalysis. A concerted metallation/deprotonation (CMD) process. Full size image Use of amino esters To show the power of this method, the protected linear amino acid esters 5 and 7 were submitted to the standard condition, and both 3-methylproline 6 and 2-tetrahydroquinonylcarboxilic ester 8 were obtained in satisfying yield. Moreover, more complicated 9 is also converted into tetrasubstituted pyrrolidine 10 as the epimer of natural (−)-codonopsinine with a sole diastereoisomer in a single operation. To our satisfaction, tricyclic scaffold 12 , containing the core structure of the natural product martinellic acid, can be also constructed via double aminations, in which both primary C sp3 –H and aromatic C Ar –H are aminated in a single operation, showing the beauty of this chemistry in organic synthesis. In conclusion, we first developed an unprecedented site-selective amination of C–H bonds without the requirement of special complicated directing groups. N -heterocyclic products bearing complex functionalities were constructed from simple and easily available linear triflamines via reliable and easily handled Ag catalysis. The method displayed unique chemo- and regioselectivities that differed from the existing methods. This study highlighted the manipulation of unfunctionalized groups in organic molecules to furnish the complex privileged structural units in the synthesis of natural products and bioactive molecules using a new pathway that is broadly applicable in organic synthesis. Materials Materials were obtained from commercial suppliers or prepared according to standard procedures unless otherwise noted. AgOAc and PhI(OTFA) 2 were purchased from J&K Chemical Co., Ltd. 4,4′-Di-tert-butyl-2,2′-dipyridyl was purchased from Sigma-Aldrich. Potassium carbonate, anhydrous (K 2 CO 3 ) was purchased from Alfa Aesar used without any further purification. All the solvents and other reagents were directly used from the purchased without any further purification unless otherwise specified. General spectroscopic methods For NMR and X-ray analysis of compounds in this paper, see Supplementary Figs 1–140 and Supplementary Tables 4–6 . NMR spectra were recorded on Bruker 400 and 500 M nuclear resonance spectrometers unless otherwise specified. CDCl 3 as solvent and tetramethylsilane (TMS) as the internal standard were employed. Chemical shift values for 1 H NMR and 13 C NMR are referenced to residual solvent peaks (CHCl 3 in CDCl 3 : 7.26 p.p.m. for 1 H, 77.00 p.p.m. for 13 C). Chemical shifts are reported in δ p.p.m. All coupling constants ( J values) were reported in Hertz (Hz). Data for 1 H NMR spectra are reported as follows: chemical shift (p.p.m., referenced to TMS; s=singlet, d=doublet, t=triplet, q=quartet, dd=doublet of doublets, dt=doublet of triplets, m=multiplet), coupling constant (Hz) and integration. 19 F NMR data was obtained on Varian 300 M nucleus resonance spectrometers. Column chromatography was performed on silica gel 200–300 mesh. HRMS (high-resolution mass spectra) were recorded on a Bruker Apex IV FTMS mass spectrometer (ESI) in the State-authorized Analytical Center at Peking University. 1 H NMR, 13 C NMR and ESI spectra are provided for all compounds. See the Supplementary Methods for the characterization data for compounds not listed in this section. Synthesis of 3-Methyl-1-(trifluoromethyl)sulfonyl-pyrrolidine 2a Silver acetate (AgOAc, 8.3 mg, 0.05 mmol), 4,4′-Di-tert-butyl-2,2′-dipyridyl (dtbpy, 13.4 mg, 0.05 mmol), [Bis(trifluoroacetoxy)iodo]benzene (PhI(OTFA) 2 , 215 mg, 0.5 mmol) and potassium carbonate (K 2 CO 3 , 69 mg, 0.5 mmol) were placed in a vial under air. Chlorobenzene (PhCl, 1.5 ml), triflamide 1a (54.8 mg, 0.25 mmol), dichloroethane (1.5 ml) were sequentially added. The mixture was stirred at room temperature for 5 min and then was stirred for 12 h at 120 °C. After the reaction mixture was cooled to room temperature, direct flash silica gel column purification (eluent: 100 ml of PE; then PE/DCM/Et 2 O 250/20/5) of the reaction solution provided 2a (40 mg, 0.17 mmol) in 70% isolated yield. (Because the boiling point of desired product is low, the solvent should be evaporated under low temperature). Colourless oil. 1 H NMR (400 MHz, CDCl 3 ) δ 3.63–3.71 (m, 2H), 3.52 (q, J =8.0 Hz, 1H), 3.06 (t, J =8.0 Hz, 1H), 2.40 (octet, J =8.0 Hz, 1H), 2.13 (sext, J =8.0 Hz, 1H), 1.65 (tq, J =8.0, 12.0 Hz, 1H), 1.11 (d, J =4.0 Hz, 3H). 13 C NMR (100 MHz, CDCl 3 ) δ 120.44 (q, J =322.0 Hz), 55.32, 48.56, 33.90, 33.57, 17.00. HRMS–ESI ( m/z ): [M+Na] + calcd for C 6 H 10 F 3 NNaO 2 S, 240.02765; found, 246.02789. Accession codes: The X-ray crystallographic structures for 9,10,12 reported in this article have been deposited at the Cambridge Crystallographic Data Centre (CCDC), under deposition number CCDC 1005416, 1005417,1005418. These data can be obtained free of charge from the Cambridge Crystallographic Data Centre via http://www.ccdc.cam.ac.uk/data_request/cif . How to cite this article: Yang, M. et al . Silver-catalysed direct amination of unactivated C–H bonds of functionalized molecules. Nat. Commun. 5:4707 doi: 10.1038/ncomms5707 (2014).